IL-21 induces IL-22 production in CD4+ T cells Interleukin (IL)-22 produced by innate lymphoid cells (ILCs) and CD4+ T cells plays an important role in host defence and mucosal homeostasis, thus it is important to investigate the mechanisms that regulate IL-22 production. We investigated the regulation IL-22 production by CD4+ T cells. Here we show that IL-21 triggers IL-22, but not IL-17 production by CD4+ T cells. STAT3, activated by IL-21, controls the epigenetic status of the il22 promoter and its interaction with the aryl hydrocarbon receptor (AhR). Moreover, IL-21 and AhR signalling in T cells control IL-22 production and the development of dextran sodium sulphate-induced colitis in ILC-deficient mice. Thus, we have identified IL-21 as an inducer of IL-22 production in CD4+ T cells in vitro and in vivo . IL-22 is a member of the IL-10 family of cytokines; cytokines in this family display homologous secondary structures and 20–30% amino acid identity [1] . IL-22 acts on non-hematopoietic cells in epithelial tissues, which express a functional IL-22 receptor composed of an heterodimer of IL-22R1 and IL-10R2 (refs 2 , 3 ). IL-22 signalling triggers the production of anti-microbial peptides and pro-inflammatory molecules, and it also promotes tissue repair by inducing epithelial cell proliferation and survival [2] , [3] . These effects of IL-22 are thought to be responsible for its important role in the control of host defence against bacterial infections, and also in limiting tissue destruction during hepatitis, colitis, graft versus host disease and thymus involution [4] , [5] , [6] , [7] , [8] , [9] . Conversely, dysregulated IL-22 signalling contributes to the pathogenesis of psoriasis, arthritis, inflammatory bowel disease (IBD) and colon cancer [10] , [11] , [12] , [13] . IL-22 is produced by cells of the innate system, particularly innate lymphoid cells (ILCs), and also by CD4+ T cells, CD8+ T cells and γδ T cells [2] , [3] . ILCs expressing the transcription factor RORγt are an important source of IL-22 in vivo [14] . Following activation with IL-23 or IL-1β, RORγt+ ILCs produce IL-22 through a mechanism controlled by the ligand-activated transcription factor aryl hydrocarbon receptor (AhR) [15] , [16] , [17] . AhR signalling is also critical for the development of ILCs, thus it has been postulated that AhR ligands in the diet or produced by commensal bacteria regulate ILC development and function [15] , [16] , [17] . However, commensal bacteria can also promote IL-22 production through AhR-independent mechanisms, for example by inducing the production of IL-1β and IL-23 by myeloid cells [18] , [19] . CD4+ T cells also produce significant amounts of IL-22. We [20] and others [21] , [22] , [23] have shown that AhR signalling regulates the production of IL-22 by Th17 cells differentiated in the presence of IL-6 and TGFβ1. Indeed, the production of IL-22 by IL-17+ CD4+ T cells has been shown to limit tissue destruction during experimental acute hepatitis [7] and IBD [8] , [24] . Although IL-22 expression is usually linked to Th17 cells [25] , human and murine CD4+ T cells that produce high amounts of IL-22 but not IL-17 have also been identified [13] , [25] , [26] , [27] , [28] . These CD4+ IL-22+ IL-17− T cells play a protective role in mucosal anti-microbial host defence [9] , [29] . Thus, considering the significant role of IL-22 produced by CD4+ T cells in host defence and mucosal barrier integrity it is important to investigate the mechanisms that regulate IL-22 production in T cells. In vitro , the activation of naïve CD4+ T cells in the presence of cytokines that trigger STAT3 activation, such as IL-6, triggers the production of IL-22 but almost no IL-17 (ref. 13 ). IL-21, a cytokine that belongs to the type I four-α-helical-bundle family of cytokines, can replace IL-6 during the differentiation of Th17 cells [30] , [31] . Thus, in this work we investigated the role of IL-21 in the differentiation of IL-22-producing CD4+ T cells. We found that IL-21 induces the differentiation of CD4+ T cells that produce IL-22, but not IL-17, by a mechanism that involves the transcription factors STAT3, AhR and RORγt. Moreover, AhR and IL-21 signalling control IL-22 production by CD4+ T cells that limit mucosal inflammation in ILC-deficient mice. Taken together, these results indicate that IL-21 signalling controls IL-22 production by T cells that limit mucosal inflammation. IL-21 induces IL-22 expression in CD4+ T cells IL-6 triggers the production of IL-22 by naïve CD4+ T cells in the absence of IL-17 production [13] . Based on the ability of IL-21 to replace IL-6 during the differentiation of Th17 cells [30] , [31] , we investigated the role of IL-21 in the differentiation of IL-22-producing CD4+ T cells. We found that the activation of naïve CD4+ T cells with antibodies to CD3 and CD28 in the presence of IL-21 results in the production of IL-22 but not IL-17 ( Fig. 1a,b ); no significant changes in IFNγ expression were detected. The production of IL-22 induced by activation with IL-21 was comparable to that observed following activation with IL-6 ( Supplementary Fig. 1a ). Moreover, in agreement with previous reports [31] , [32] we found that exogenous IL-21 also upregulated its own expression in T cells ( Fig. 1c ), suggesting that a positive feed forward loop stabilizes IL-22 production in IL–21-stimulated T cells. The upregulation of il21 expression was reduced by TGFβ1 blockade, suggesting that it is boosted by trace amounts of TGFβ1 provided either by the medium or the T cells ( Supplementary Fig. 1b ). 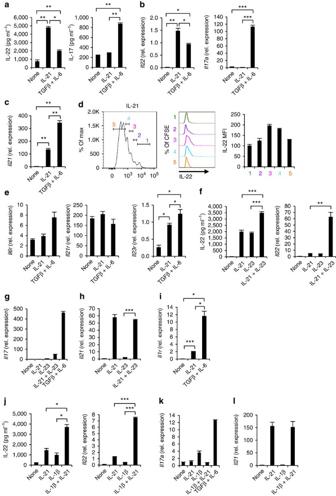Figure 1: IL-21 promotes the differentiation of CD4+ T cells that produce IL-22 but not IL-17. Naïve WT CD4+ T cells were stimulatedin vitrowith antibodies to CD3 and CD28 in the presence of different cytokines as indicated. (a,b) Effect of IL-21 in the production of IL-22 and IL-17 measured by ELISA in culture supernatants (a) and qPCR (b). (c) Effect of IL-21 on the expression ofil21. (e) Effect of IL-21 on the expression ofil6r,il21randil23r. (d) Relationship between cell division and IL-22 expression in CD4+ T cells. Carboxyfluorescein succinimidyl ester-labelled naïve CD4+ T cells were activated in the presence of IL-21 and the production of IL-22 was analysed by intracellular staining. The data are shown as the mean fluorescence intensity (MFI) for IL-22 for each division cycle. (e) Effects of IL-21 on the expression ofil6r,il21randil23r. (f–h) Synergistic effects of IL-21 and IL-23 on IL-22 (f) and IL-17 (g) cytokine andil21expression (h). (i) Effect of IL-21 onil1rexpression. (j–l) Synergistic effects of IL-21 and IL-1β on IL-22 (j),Il17a(k) andil21(l) expression. mRNA expression is shown relative togapdh. Results are representative of 3–5 independent experiments. *P<0.05, **P<0.01 and ***P<0.001 (one-way ANOVA). Figure 1: IL-21 promotes the differentiation of CD4+ T cells that produce IL-22 but not IL-17. Naïve WT CD4+ T cells were stimulated in vitro with antibodies to CD3 and CD28 in the presence of different cytokines as indicated. ( a , b ) Effect of IL-21 in the production of IL-22 and IL-17 measured by ELISA in culture supernatants ( a ) and qPCR ( b ). ( c ) Effect of IL-21 on the expression of il21 . ( e ) Effect of IL-21 on the expression of il6r , il21r and il23r . ( d ) Relationship between cell division and IL-22 expression in CD4+ T cells. Carboxyfluorescein succinimidyl ester-labelled naïve CD4+ T cells were activated in the presence of IL-21 and the production of IL-22 was analysed by intracellular staining. The data are shown as the mean fluorescence intensity (MFI) for IL-22 for each division cycle. ( e ) Effects of IL-21 on the expression of il6r , il21r and il23r . ( f – h ) Synergistic effects of IL-21 and IL-23 on IL-22 ( f ) and IL-17 ( g ) cytokine and il21 expression ( h ). ( i ) Effect of IL-21 on il1r expression. ( j – l ) Synergistic effects of IL-21 and IL-1β on IL-22 ( j ), Il17a ( k ) and il21 ( l ) expression. mRNA expression is shown relative to gapdh . Results are representative of 3–5 independent experiments. * P <0.05, ** P <0.01 and *** P <0.001 (one-way ANOVA). Full size image The production of IL-22 by T cells activated in the presence of IL-21 was associated to proliferation, peaking at three cell divisions as determined by staining with carboxyfluorescein succinimidyl ester ( Fig. 1d ). To investigate the stability of IL-22-producing T cells induced with IL-21, naïve CD4+ T cells were initially activated in the presence of IL-21, rested and reactivated in the presence of IL-21, or under Th17 (IL-6 and TGFβ1) or FoxP3 iTreg (TGFβ1)-polarizing conditions. The re-stimulation of T cells that have been previously activated in the presence of IL-21 resulted in a significant population of IL-17− IL-22+ T cells; similar results were found upon reactivation in the presence of IL-21 ( Supplementary Fig. 2c ). Re-stimulation under Th17-polarizing conditions resulted in similar numbers of IL-17− IL-22+ T cells; however, under these experimental conditions we also detected the generation of IL-17-producing T cells (IL-17+ IL-22+ and IL-17+ IL-22− T cells) ( Supplementary Fig. 2c ). Similar results were obtained following reactivation under FoxP3 iTreg-polarizing conditions, probably as a result of the promotion of Th17 cell differentiation by exogenous TGFβ1 acting in combination with T-cell-produced IL-21 (refs 30 , 31 ; Supplementary Fig. 2c ). These results suggest that IL-22-producing T cells induced with IL-21 are relatively stable, and that additional Th17 cells can be differentiated from non-polarized T cells in the culture. Since IL-6 and IL-23 have also been shown to trigger the production of IL-22 by CD4+ T cells [9] , [13] , [28] , [29] , we studied the effects of IL-21 on the expression of IL-6R, IL-23R and IL-21R. T-cell activation in the presence of IL-21 resulted in a significant upregulation of il23r expression, but did not modify the expression of il6r or il21r ( Fig. 1e ), suggesting that IL-21 signalling may also modulate the production of IL-22 triggered in CD4+ T cells by IL-23. Similar levels of il21r and il23r expression were observed following T-cell stimulation in the presence of IL-21 or IL-6 ( Supplementary Fig. 1d ). In accordance with these findings, we found a significant synergism between IL-21 and IL-23 in inducing IL-22 expression in CD4+ T cells ( Fig. 1f,g ). IL-23, however, did not synergize with IL-21 to boost il21 expression by T cells ( Fig. 1h ). IL-1β boosts IL-22 production by Th17 cells [33] , thus we investigated the effects of IL-1β in the production of IL-22 triggered by IL-21. We found that IL-21 upregulated il1r1 expression in T cells; this upregulation was partially dependent on TGFβ1 signalling ( Fig. 1i and Supplementary Fig. 1d ). Moreover, IL-1β synergized with IL-21 in inducing the production of IL-22, but not that of IL-17 ( Fig. 1j,k ). IL-1β, however, did not boost il21 expression induced by IL-21 ( Fig. 1l ). Taken together, these results suggest that IL-21, alone or in combination with IL-23 or IL-1β, triggers IL-22 production independently of IL-17 in CD4+ T cells. Transcriptional profiling of IL-21-stimulated CD4+ T cells To study the molecular mechanisms mediating the production of IL-22 by CD4+ T cells stimulated with IL-21, we analysed the mRNA expression profile by whole-genome microarrays. We compared the mRNA expression profiles of naïve CD4+ T cells activated in the presence of IL-21, IL-6 and TGFβ1 (Th17 cells) or without the addition of exogenous cytokines (Th0 cells). We found 869 genes that were up- or downregulated at least 1.5-fold in CD4+ T cells stimulated in the presence of IL-21 relative to their expression in control Th0 cells ( Fig. 2a ). Principal component analysis showed that the transcriptional signature of CD4+ T cells treated with IL-21 is significantly different from that of Th17 cells differentiated with IL-6 and TGFβ1 ( Fig. 2b ). Although there was a partial overlap between genes upregulated in IL-22+ IL-17− T cells and Th17 cells, a direct comparison of their transcriptional profile identified 179 genes with differences in expression. We found significant differences in the expression of key cytokines, chemokines, receptors and transcription factors recently associated with Th17 cells differentiated in vitro with TGFβ1 and IL-6 (ref. 34 ; Fig. 2c ). We focused our attention on transcriptional modules recently identified to control Th17 cell differentiation: a module of ‘Th17-positive factors’ that promote Th17 cell differentiation and a module of ‘Th17-negative factors’ that interferes with this process [34] . We found that IL-22-producing T cells induced with IL-21 differed from Th17 cells in the expression of genes belonging to these Th17-positive and Th17-negative transcriptional modules ( Fig. 2d ). 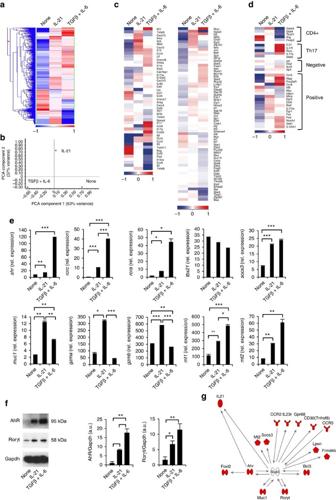Figure 2: Transcriptional profiling of IL-21-stimulated CD4+ T cells. Naïve WT CD4+ T cells were stimulatedin vitrowith antibodies to CD3 and CD28 in the presence of IL-21, IL-6 and TGFβ1 or without addition of exogenous cytokines. (a) Heat map showing genes with at least a 1.5-fold change in expression relative to Th0 as determined by whole-genome microarrays. (b) Principal component analysis. (c,d) Heat maps depicting the expression of key cytokines, chemokines, receptors and transcription factors (c) and transcriptional modules (d) that control the differentiation of Th17 cells as defined in ref.34. (e) Quantitative RT–PCR analysis of the expression of genes inFig. 2a. mRNA expression is shown relative togapdh. (f) Western blot analysis of the expression of AhR (95 kDa) and RORγt (58 kDa) on T cells activated in the presence of IL-21 or under Th17-polarizing conditions (left panel). Quantification of western blot reactivity (right panel). (g) Ingenuity pathways analysis of the transcriptional response of naïve CD4+ T cells to IL-21. *P<0.05, **P<0.01 and ***P<0.001 (one-way ANOVA). Figure 2: Transcriptional profiling of IL-21-stimulated CD4+ T cells. Naïve WT CD4+ T cells were stimulated in vitro with antibodies to CD3 and CD28 in the presence of IL-21, IL-6 and TGFβ1 or without addition of exogenous cytokines. ( a ) Heat map showing genes with at least a 1.5-fold change in expression relative to Th0 as determined by whole-genome microarrays. ( b ) Principal component analysis. ( c , d ) Heat maps depicting the expression of key cytokines, chemokines, receptors and transcription factors ( c ) and transcriptional modules ( d ) that control the differentiation of Th17 cells as defined in ref. 34 . ( e ) Quantitative RT–PCR analysis of the expression of genes in Fig. 2a . mRNA expression is shown relative to gapdh . ( f ) Western blot analysis of the expression of AhR (95 kDa) and RORγt (58 kDa) on T cells activated in the presence of IL-21 or under Th17-polarizing conditions (left panel). Quantification of western blot reactivity (right panel). ( g ) Ingenuity pathways analysis of the transcriptional response of naïve CD4+ T cells to IL-21. * P <0.05, ** P <0.01 and *** P <0.001 (one-way ANOVA). Full size image On the basis of the biological function of their products, we selected a representative subset of genes coding for transcription factors such as ahr , rora , rorc , tbx21 and socs3 ; granzymes A and B ( gzma and gzmb ), which have been linked to effector and regulatory T cells [35] ; the IBD-linked mucin 1 ( muc1 ), known to be a transcriptional target of STAT3 (refs 36 , 37 , 38 ), and the inhibitors of IL-10 production metallothioneins 1 and 2 ( mt1 and mt2 ) [34] and confirmed their differences in expression by qPCR ( Fig. 2e ). The upregulation of AhR and RORγt expression was also confirmed at the protein level by western blot ( Fig. 2f ). However, and in agreement with previous reports on IL-22-producing T cells generated with IL-6 (ref. 28 ), this upregulation was promoted by trace amounts of TGFβ1 provided either by the medium or the T cells, because it could be inhibited with TGFβ1-specific blocking antibodies ( Supplementary Fig. 2a ). Of note, activation of T cells in the presence of IL-21 did not result in a significant upregulation of tbx21 , which has been recently linked to the production of IL-22 triggered in CD4+ T cells IL-6 (ref. 29 ). We also failed to detect foxp3 expression in T cells activated in the presence of IL-21 ( Supplementary Fig. 2b ). Finally, we used Ingenuity Pathways Analysis to analyse the genes found to be differentially expressed between Th0 and IL-22+ IL-17− T cells. The resulting model identified important roles for STAT3, RORγt and AhR in the control of IL-22+ IL-17− T cell differentiation triggered by IL-21 ( Fig. 2g ). In conclusion, these data suggest that IL-21 triggers a transcriptional programme in CD4+ T cells that differs from the one of Th17 cells and is controlled by STAT3, RORγt and AhR. STAT3 is required for IL-21-induced IL-22 expression Based on our transcriptional analysis and the reported activation of STAT3 by IL-21 signalling, we studied the role of STAT3 in the production of IL-22 triggered by IL-21. T-cell activation in the presence of IL-21 led to a significant phosphorylation of STAT3, and also to a significant increase in stat3 expression ( Fig. 3a,b ). T-cell activation in the presence of IL-6, with or without TGFβ1-blocking antibodies, resulted in similar amounts of STAT3 phosphorylation ( Supplementary Fig. 3a ). 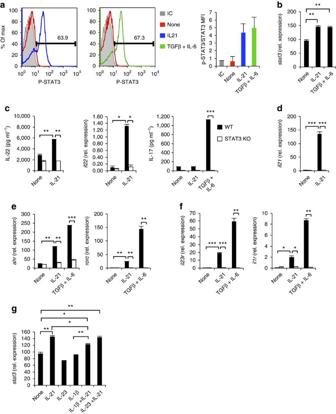Figure 3: STAT3 controls the production of IL-22 by CD4+ T cells stimulated with IL-21. (a,b) Naïve WT CD4+ T cells were activated in the presence of IL-21 or IL-6 and TGFβ1. (a) FACS analysis of phosphorylated STAT3. Mean fluorescence intensity (MFI) of phosphorylated STAT3 normalized to total STAT3. (b) qPCR analysis ofstat3expression. (c–f) Naïve WT and STAT3-deficient CD4+ T cells were activated in the presence of IL-21 or IL-6 and TGFβ1. (c) Effect of STAT3 deficiency on IL-22 and IL-17 production. (d) Effect of STAT3 deficiency onil21expression. (e,f) Effect of STAT3 deficiency onahrandrorcexpression (e) and the receptorsil1randil23r(f). (g) Induction ofstat3by IL-1β, IL-21, IL-23, IL-1β and IL-21 or IL-21 and IL-23. mRNA expression is shown relative togapdh. Results are representative of two to three independent experiments. *P<0.05, **P<0.01 and ***P<0.001 (one-way ANOVA and Student’st-test). Figure 3: STAT3 controls the production of IL-22 by CD4+ T cells stimulated with IL-21. ( a , b ) Naïve WT CD4+ T cells were activated in the presence of IL-21 or IL-6 and TGFβ1. ( a ) FACS analysis of phosphorylated STAT3. Mean fluorescence intensity (MFI) of phosphorylated STAT3 normalized to total STAT3. ( b ) qPCR analysis of stat3 expression. ( c – f ) Naïve WT and STAT3-deficient CD4+ T cells were activated in the presence of IL-21 or IL-6 and TGFβ1. ( c ) Effect of STAT3 deficiency on IL-22 and IL-17 production. ( d ) Effect of STAT3 deficiency on il21 expression. ( e , f ) Effect of STAT3 deficiency on ahr and rorc expression ( e ) and the receptors il1r and il23r ( f ). ( g ) Induction of stat3 by IL-1β, IL-21, IL-23, IL-1β and IL-21 or IL-21 and IL-23. mRNA expression is shown relative to gapdh . Results are representative of two to three independent experiments. * P <0.05, ** P <0.01 and *** P <0.001 (one-way ANOVA and Student’s t -test). Full size image To investigate the function of STAT3 in the regulation of IL-22 production, we activated wild type (WT) and STAT3-deficient CD4+ T cells in the presence of IL-21. The production of IL-22 in response to IL-21 was significantly decreased in STAT3-deficient CD4+ T cells ( Fig. 3c ). Moreover, in agreement with our bioinformatic analysis STAT3 was also required for the upregulation of il21 , ahr and rorc expression in response to IL-21 ( Fig. 3d,e ). Of note, we also found that STAT3 mediated the upregulation of il23r and il1r1 expression in response to IL-21 ( Fig. 3f ). However, IL-23 or IL-1β did not upregulate stat3 expression when their effects on CD4+ T cells were analysed alone or in combination with IL-21 ( Fig. 3g ). Taken together, these data suggest that STAT3 plays a central role in the differentiation of IL-22-producing CD4+ T cells in response to IL-21. RORγt and AhR control IL-22 expression induced by IL-21 The upregulation of rorc expression was linked to the induction of IL-22 expression in CD4+ T cells triggered by IL-21 ( Fig. 2 ). Based on our studies on the transcriptional effects of IL-21 on CD4+ T cells and the reported role of RORγt in the control of il22 expression in Th17 cells and ILCs [16] , [39] we investigated the role of RORγt in the production of IL-22 triggered by IL-21. We found that RORγt deficiency led to a significant reduction in the production of IL-22 induced by IL-21 in naïve CD4+ T cells ( Fig. 4a ). RORγt deficiency also decreased the expression of il23r but not of il1r1 , and abrogated the ability of IL-23 to boost IL-22 production triggered by IL-21 ( Fig. 4b,c ). Conversely, activation of naïve T cells in the presence of IL-23 or IL-1β alone did not result in a significant upregulation of rorc expression, but IL-23 synergized with IL-21 to boost rorc expression ( Fig. 4d ). Thus, similarly to what has been described for Th17 cells and ILCs, RORγt controls the production of IL-22 by CD4+ T cells treated with IL-21. Moreover, these data suggest that in addition to its effects on the production of IL-22 triggered by IL-21, RORγt also controls the ability of IL-23 to synergize with IL-21 and boost IL-22 expression in T cells. 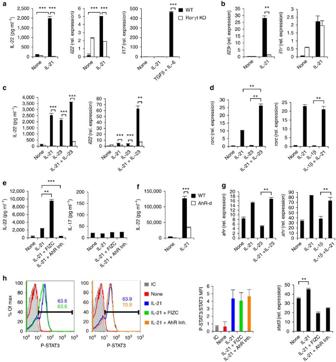Figure 4: RORγt and AhR control IL-22 production by CD4+ T cells stimulated with IL-21. (a–c) Naïve WT and RORγt-deficient CD4+ T cells were activated in the presence of IL-21 or IL-6 and TGFβ1. (a) Effect of RORγt deficiency on IL-22 and IL-17 production. (b) Effect of RORγt deficiency onil23randil1r1expression. (c) Effect of RORγt deficiency on the synergism between IL-21 and IL-23. (d) Effect of IL-1β and IL-23 inrorcexpression. (e) Effect of the modulation of AhR activity on IL-22 and IL-17 production. (f) IL-22 production by WT and AhR-d CD4+ T cells activated in the presence of IL-21. (g) Modulation ofahrexpression by IL-1β and IL-23. (h) Effect of AhR modulation on STAT3 phosphorylation andstat3expression. MFI of phosphorylated STAT3 normalized to total STAT3. mRNA expression is shown relative togapdh. Representative results of two to three independent experiments. **P<0.01 and ***P<0.001 (one-way ANOVA and Student’st-test). Figure 4: RORγt and AhR control IL-22 production by CD4+ T cells stimulated with IL-21. ( a – c ) Naïve WT and RORγt-deficient CD4+ T cells were activated in the presence of IL-21 or IL-6 and TGFβ1. ( a ) Effect of RORγt deficiency on IL-22 and IL-17 production. ( b ) Effect of RORγt deficiency on il23r and il1r1 expression. ( c ) Effect of RORγt deficiency on the synergism between IL-21 and IL-23. ( d ) Effect of IL-1β and IL-23 in rorc expression. ( e ) Effect of the modulation of AhR activity on IL-22 and IL-17 production. ( f ) IL-22 production by WT and AhR-d CD4+ T cells activated in the presence of IL-21. ( g ) Modulation of ahr expression by IL-1β and IL-23. ( h ) Effect of AhR modulation on STAT3 phosphorylation and stat3 expression. MFI of phosphorylated STAT3 normalized to total STAT3. mRNA expression is shown relative to gapdh . Representative results of two to three independent experiments. ** P <0.01 and *** P <0.001 (one-way ANOVA and Student’s t -test). Full size image We [20] and others [21] , [22] , [23] found that AhR activation modulates IL-22 production in Th17 cells. Moreover, AhR also participates in the production of IL-22 triggered by IL-6 (ref. 28 ). Based on these observations and the results of our transcriptional profiling of CD4+ T cells activated in the presence of IL-21 ( Fig. 2 ), we investigated the role of AhR in the control of IL-22 production triggered by IL-21. The addition of the AhR agonist 6-formylindolo[3,2-b]carbazole (FICZ) led to a significant increase in the production of IL-22 triggered by IL-21 ( Fig. 4e ). Conversely, the use of the AhR-specific antagonist CH-223191 resulted in a significant reduction in IL-22 production triggered by IL-21 ( Fig. 4e ). A similar reduction in IL-22 production was detected when we used T cells from AhR-d mice, which carry an ahr allele coding for a mutant AhR with reduced affinity for its ligands [40] ; ( Fig. 4f ). Of note, ahr expression levels were not significantly upregulated in response to T-cell activation in the presence of IL-23 or IL-1β alone, and IL-23 or IL-1β did not synergize with IL-21 to upregulate ahr expression ( Fig. 4g ). These findings suggest that AhR plays a more important role in the regulation of IL-22 production by CD4+ T cells activated by IL-21 than in response to IL-23 or IL-1β. AhR has been shown to interact with STAT proteins and modulate their activity [21] , [22] , [41] . Considering the important role of STAT3 in the production of IL-22 triggered by IL-21, we analysed whether STAT3 activation in response to IL-21 is modulated by AhR. We found that modulation of AhR signalling with FICZ or CH-223191 had no significant effect in the phosphorylation of STAT3 in T cells in response to IL-21 ( Fig. 4h ). Similarly, we found no significant differences in STAT3 phosphorylation in response to IL-21 between WT and AhR-d T cells ( Supplementary Fig. 3b ). Taken together, these data suggest that RORγt and AhR control the IL-22 production triggered by IL-21, and these effects do not involve the modulation of STAT3 activation. STAT3 controls the accessibility of the il22 promoter We recently reported that AhR and STAT3 co-operate to regulate ikzf3 expression in Th17 cells [42] . A bioinformatic analysis of the il22 promoter revealed two putative STAT3 responsive elements (SRE-1 and SRE-2) upstream of the transcription start site and three putative binding sites for AhR (xenobiotic response elements, XRE-1, XRE-2 and XRE-3) ( Fig. 5a ). Thus, to investigate whether STAT3 and AhR interact with these potential binding sites in the il22 locus we performed chromatin immunoprecipitation (ChIP) assays. We detected a significant interaction of AhR and STAT3 with the il22 promoter in CD4+ T cells activated in the presence of IL-21 ( Fig. 5b,c ). 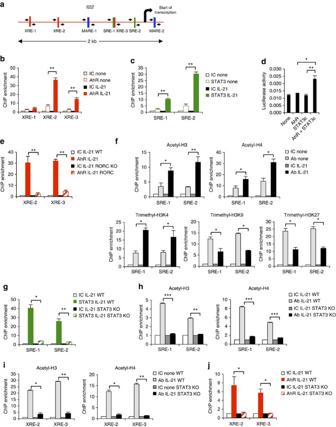Figure 5: STAT3 controls AhR recruitment to theil22promoter in IL-21-stimulated CD4+ T cells. (a) AhR, c-Maf and STAT3 binding sites in theil22promoter. (b,c) WT naïve CD4+ T cells were stimulatedin vitrowith antibodies to CD3 and CD28 in the presence or absence of IL-21. ChIP analysis of the interaction of AhR (b) and STAT3 (c) to the AhR- and STAT3-binding sites in theil22promoter, respectively. (d) Regulation of the transcriptional activity of theil22promoter by AhR and STAT3. A reporter construct for theil22promoter (il22:Luc) was cotransfected in HEK293 cells with vector coding for AhR and/or constitutively activated STAT3 (STAT3c). Firefly luciferase was determined and normalized to renilla luciferase activity. (e) ChIP analysis of the recruitment of AhR to theil22promoter in WT and RORγt-deficient CD4+ cells activated in the presence of IL-21. (f) WT naïve CD4+ T cells were stimulatedin vitrowith antibodies to CD3 and CD28 in the presence or absence of IL-21, and the epigenetic status of theil22promoter was analysed by ChIP using antibodies to Acetyl-H3, Acetyl-H4 and H3 trimethylated at Lys4, Lys9 or Lys27. (g–j) ChIP analysis of the epigenetic status of theil22promoter in WT and STAT3-deficient CD4+ T cells activated in the presence of IL-21. STAT3 recruitment (g), H3 and H4 acetylation in SREs (h) and XREs (i) and AhR recruitment (j) in theil22promoter. Results are representative of two to three independent experiments. *P<0.05, **P<0.01 and ***P<0.001 (one-way ANOVA). Figure 5: STAT3 controls AhR recruitment to the il22 promoter in IL-21-stimulated CD4+ T cells. ( a ) AhR, c-Maf and STAT3 binding sites in the il22 promoter. ( b , c ) WT naïve CD4+ T cells were stimulated in vitro with antibodies to CD3 and CD28 in the presence or absence of IL-21. ChIP analysis of the interaction of AhR ( b ) and STAT3 ( c ) to the AhR- and STAT3-binding sites in the il22 promoter, respectively. ( d ) Regulation of the transcriptional activity of the il22 promoter by AhR and STAT3. A reporter construct for the il22 promoter (il22:Luc) was cotransfected in HEK293 cells with vector coding for AhR and/or constitutively activated STAT3 (STAT3c). Firefly luciferase was determined and normalized to renilla luciferase activity. ( e ) ChIP analysis of the recruitment of AhR to the il22 promoter in WT and RORγt-deficient CD4+ cells activated in the presence of IL-21. ( f ) WT naïve CD4+ T cells were stimulated in vitro with antibodies to CD3 and CD28 in the presence or absence of IL-21, and the epigenetic status of the il22 promoter was analysed by ChIP using antibodies to Acetyl-H3, Acetyl-H4 and H3 trimethylated at Lys4, Lys9 or Lys27. ( g – j ) ChIP analysis of the epigenetic status of the il22 promoter in WT and STAT3-deficient CD4+ T cells activated in the presence of IL-21. STAT3 recruitment ( g ), H3 and H4 acetylation in SREs ( h ) and XREs ( i ) and AhR recruitment ( j ) in the il22 promoter. Results are representative of two to three independent experiments. * P <0.05, ** P <0.01 and *** P <0.001 (one-way ANOVA). Full size image We then analysed the functional effects of the interaction of STAT3 and AhR with its DNA responsive elements using a reporter plasmid carrying the firefly luciferase under the control of the il22 promoter (il22:Luc). Transfection with vectors coding for AhR or constitutively activated STAT3 did not result in a significant induction of luciferase activity ( Fig. 5d ). However, co-transfection with constructs coding for constitutively activated STAT3 and AhR induced a significant upregulation of luciferase activity, suggesting a synergistic effect of STAT3 and AhR in the production of IL-22 ( Fig. 5d ). c-Maf interacts with AhR to transactivate the il10 promoter [35] , [43] , but it suppresses il22 expression induced with IL-6 (ref. 28 ). Although we detected a small upregulation of maf in response to IL-21 ( Supplementary Fig. 4a ), we found no significant binding of c-Maf to its potential binding sites in the il22 promoter ( Supplementary Fig. 4b ). These data suggest that, similarly to what has been described for IL-22+ IL-17- T cells induced with IL-6, c-Maf does not promote il22 expression in T cells activated in the presence of IL-21 (ref. 28 ). Both AhR and RORγt have been shown to control IL-22 expression in Th17 cells. Indeed, AhR and RORγt physically interact, and in overexpression experiments in EL4 cells it was shown that a constitutively active mutant AhR is recruited to the il22 locus in a RORγt-dependent manner [16] . Since we found that RORγt-deficient T cells show a significant decrease in IL-22 production following activation in the presence of IL-21, we investigated whether RORγt was needed for the recruitment of endogenous AhR to its target sequences in the il22 locus. We found that RORγt deficiency results in a significant decrease in the recruitment of AhR to the il22 promoter ( Fig. 5e ). We also detected a decrease in the acetylation of histones 3 and 4 and the trimethylation of histone 3 at Lys4, concomitant with increased histone trimethylation at Lys9 and Lys27, supporting our findings on the lack of il22 expression in the absence of RORγt ( Supplementary Fig. 4c ). Overexpression of AhR and RORγt in CD4+ T cells activated under non-polarizing Th0 conditions, however, does not result in IL-22 expression [22] . The ability of transcription factors to bind regulatory regions on target genes is affected by the structure of the chromatin, which is regulated by several processes including post-translational histone modifications [44] . Thus, we reasoned that the lack of IL-22 expression observed in CD4+ T cells overexpressing AhR and RORγt (ref. 22 ) might reflect the need for epigenetic mechanisms that increase the accessibility to regulatory elements in the il22 promoter. First, we analysed the acetylation status of histone H3 and H4 in the il22 promoter of naïve T cells activated in the presence of IL-21. We found a significant increase in the acetylation of histones H3 and H4 in CD4+ T cells activated in the presence of IL-21 ( Fig. 5f ), which is usually associated with a relaxed chromatin structure that facilitates the interaction of transcription factors with target sequences. We also found that T-cell activation in the presence of IL-21 results in increased histone 3 trimethylation in Lys4, associated to actively transcribed genes, concomitant with decreased trimethylation in Lys9 and Lys27, which have been associated with the silencing of transcription [45] ( Fig. 5f ). Of note, we detected no changes in the methylation status of the il22 promoter ( Supplementary Fig. 4d ). STAT3 binds target sequences in the il22 promoter and is required for the production of IL-22 triggered by IL-21 ( Figs 3c and 5c ). Given the reported role of STAT3 in regulating the epigenetic status of target genes [46] , we investigated the role of STAT3 in regulating the epigenetic status of the il22 locus using WT and STAT3-deficient T cells activated in the presence of IL-21. We found that the lack of STAT3 recruitment to the il22 promoter in STAT3-deficient T cells resulted in a significant decrease in H3 and H4 acetylation in STAT3 and AhR binding sites ( Fig. 5g–i ). We also detected a decrease in histone 3 trimethylation at Lys4 and an increase in trimethylation at Lys9 and Lys27 in STAT3-deficient T cells ( Supplementary Fig. 4e ). Moreover, the reduced histone acetylation observed in STAT3-deficient T cells was concomitant with a reduced recruitment of AhR to the il22 promoter ( Fig. 5j ). Taken together, these results demonstrate that in addition to its effects on the expression of AhR and RORγt, STAT3 activated in response to IL-21 controls the accessibility to regulatory elements in the il22 promoter recognized by AhR and probably additional transcription factors. IL-21 and AhR control IL-22 expression in vivo IL-22 maintains the integrity of the colonic epithelium during inflammation [8] , [24] . Dextran sodium sulphate (DSS)-induced colitis is thought to result from the disruption of the epithelial barrier in the colon, resulting in the translocation of commensal bacteria, the activation of innate immunity and upregulation of IL-23 and IL-6 (ref. 47 ). IL-22 plays a central role in the control of intestinal inflammation [2] , [3] . Although both ILCs and CD4+ T cells produce IL-22 during the course of DSS-induced colitis, ILCs constitute a more abundant source of IL-22 in WT mice ( Supplementary Fig. 5 ). The development of ILCs is regulated by IL-7 signalling through the IL-2 receptor common gamma chain (IL-2RG) [48] . Thus, to focus our studies on the role of IL-22-producing CD4+ T cells during gut inflammation, we used mice deficient in both RAG2 and IL-2RG (RAG2/IL2RG mice); these mice lack T cells and also NK cells and ILCs [3] , [17] . To study the role of AhR and IL-21 in the regulation of IL-22 production by T cells in vivo , we reconstituted RAG2/IL2RG mice with WT CD4+ T cells, IL-21R-deficient (IL-21R KO) T cells or AhR-d T cells. Following confirmation of successful T-cell reconstitution by flow cytometry from blood samples, we induced DSS colitis in the recipient mice and monitored weight change daily. We found a significant worsening of DSS-induced colitis in mice reconstituted with AhR-d or IL-21R-deficient T cells, manifested as increased weight loss ( Fig. 6a ) and colon shortening ( Fig. 6b ), suggestive of augmented colon inflammation. Accordingly, IL-21R KO and AhR-d mice showed increased colon inflammation upon blind histological examination ( Fig. 6c ). 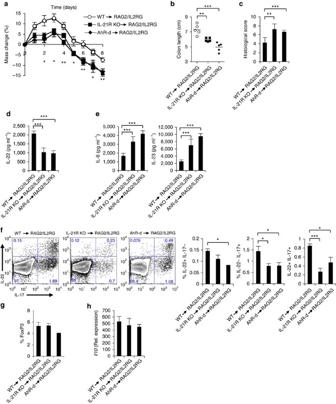Figure 6: IL-21 and AhR control IL-22+ CD4+ T cellsin vivoand limit mucosal inflammation. (a) RAG2/IL2RG mice transferred with WT, AhR-d or IL-21R-deficient CD4+ T cells were given 3% DSSad libitumin their drinking water for 7 days. Body weight was assessed daily, and the per cent mass change from day 0 was calculated. Mean±s.e.m. is shown,n=5 mice per group. Effect of genotype on disease courseP<0.0001, *P<0.01 by two-way ANOVA. (b) Colon length at day 7 after treatment with DSS. (c) Colonic histological sections were scored as described in Methods. Values are mean±s.e.m. (d,e) Colons were excised on day 7 after the initiation of treatment with DSS, cultured for 3 days and IL-22 (d), IL-6 and IL-23 (e) were quantified in the supernatants by ELISA. (f–h) Lymphocytes from the colonic lamina propria (LPL) were isolated. The frequency of IL-22+IL17−, IL-22+IL-17+, IL-22−IL-17+ T cells (f) and FoxP3+ Tregs (g) was analysed by FACS and the expression ofil10was measured by qPCR (h). mRNA expression is shown relative to the expression ofgapdh.Results are representative of three independent experiments. *P<0.05, **P<0.01 and ***P<0.001 (one-way ANOVA and two-way ANOVA). Figure 6: IL-21 and AhR control IL-22+ CD4+ T cells in vivo and limit mucosal inflammation. ( a ) RAG2/IL2RG mice transferred with WT, AhR-d or IL-21R-deficient CD4+ T cells were given 3% DSS ad libitum in their drinking water for 7 days. Body weight was assessed daily, and the per cent mass change from day 0 was calculated. Mean±s.e.m. is shown, n =5 mice per group. Effect of genotype on disease course P< 0.0001, * P< 0.01 by two-way ANOVA. ( b ) Colon length at day 7 after treatment with DSS. ( c ) Colonic histological sections were scored as described in Methods. Values are mean±s.e.m. ( d , e ) Colons were excised on day 7 after the initiation of treatment with DSS, cultured for 3 days and IL-22 ( d ), IL-6 and IL-23 ( e ) were quantified in the supernatants by ELISA. ( f – h ) Lymphocytes from the colonic lamina propria (LPL) were isolated. The frequency of IL-22+IL17−, IL-22+IL-17+, IL-22−IL-17+ T cells ( f ) and FoxP3+ Tregs ( g ) was analysed by FACS and the expression of il10 was measured by qPCR ( h ). mRNA expression is shown relative to the expression of gapdh. Results are representative of three independent experiments. * P <0.05, ** P <0.01 and *** P <0.001 (one-way ANOVA and two-way ANOVA). Full size image To directly investigate the impact of IL-21 and AhR signalling in T cells on the immune response during DSS-induced colitis, we analysed cytokine production by excised colon cultures prepared from mice reconstituted with WT, AhR-d or IL-21R-deficient T cells. We found a significant reduction in the production of IL-22 by colon explants isolated from AhR-d or IL-21R-deficient mice ( Fig. 6d ) and a concomitant increase in the levels of the pro-inflammatory cytokines IL-6 and IL-23 ( Fig. 6e ). The decreased production of IL-22 correlated with a decrease in the frequency of IL-22-producing T cells in AhR-d and IL21R-deficient mice compared with WT ( Fig. 6f ). Of note, we did not detect significant changes in il10 expression nor in the frequency of FoxP3+ T cells ( Fig. 6g ). Taken together, these results demonstrate that IL-21 and AhR signalling in T cells limit gut inflammation. IL-22 regulates tissue homeostasis and inflammation at mucosal surfaces [2] , [3] . ILCs have been identified as an important source of IL-22 in vivo , but the importance of IL-22-producing T cells and the mechanisms regulating their differentiation and function are largely unknown. Human and murine γδ T cells, Th1 and Th17 cells produce IL-22 (refs 2 , 3 ). In addition, IL-22+ IL-17- cells named Th22 cells have been described in humans [26] , [27] but it has proven difficult to identify the murine equivalent of this population. CD4+ T-cell activation in the presence of IL-6, IL-21 or IL-23 induces IL-22+ IL-17− T cells that have been linked to early host defence against Citrobacter rodentium [9] , [13] , [28] , [29] , [49] . Activation of Notch signalling has also been shown to induce IL-22 production by CD4+ T cells in a STAT3-independent manner [50] . These data suggest that, similarly to what is observed for human Th22 cells, IL-22 can be expressed independently of IL-17 in mouse T cells. However, until specific transcription factors are identified to act as master regulators of IL-22+ IL-17− T cells, it cannot be determined whether these cells constitute a separate CD4+ T cell lineage or simply represent an activation stage of CD4+ T cells. IL-21 is produced by NKT cells, γδ T cells, follicular helper T cells, Th17 cells, type 1 regulatory T cells and a recently described subpopulation of mucosal CCR9+ Th cells [43] , [51] . Thus, these cell populations may regulate the production of IL-21-dependent IL-22 by T cells in vivo . We found that IL-21 upregulates rorc expression, and also il1r1 and il23r in a RORγt-dependent manner. Indeed, IL-21 synergized with IL-1β and IL-23 to induce IL-22 production by CD4+ T cells. These data suggest that by increasing il1r1 and il23r expression, IL-21 decreases the activation threshold for IL-1β and IL-23-triggered IL-22 production. In addition, IL-6 has also been shown to induce IL-21 production by T cells [32] . Thus, it is likely that similarly to their reported effects on Th17 cell differentiation [52] , IL-21 acts in combination with IL-23, IL-1β and IL-6 to stabilize and boost the production of IL-22 by T cells in vivo . IL-21 can replace IL-6 during the differentiation of Th17 cells, and IL-21 and IL-6 exhibit redundancy during the differentiation of follicular T helper cells [30] , [31] , [51] ; however, that redundancy is not complete in vivo [53] . Future studies should determine the relative contribution of IL-6 and IL-21, and also IL-1β and IL-23 during the regulation of IL-22 production by T cells and other cell populations. Group 3 ILCs comprises an heterogeneous group of cell populations identified as a major source of IL-22 in vivo [2] , [14] , [24] . Interestingly, AhR and RORγt are reported to control IL-22 production by ILCs in response to IL-23, a known activator of STAT3 signalling [15] , [16] . These reports and the data presented in this manuscript highlight the transcriptional similarities existing between CD4 T cells activated in the presence of IL-21 and group 3 ILCs, and suggest that additional transcriptional elements involved in the control of IL-22 expression might be shared by these two sources of IL-22. Of note, it has been recently shown that T-bet controls the production of IL-22 production triggered with IL-6 (ref. 29 ). In our experiments we did not detect an upregulation of tbx21 following T-cell activation in the presence of IL-21. This finding suggests that similarly to the heterogeneity that characterizes the RORγt+ IL-22+ cells included in group 3 ILCs, distinct IL-22+ IL-17− CD4+ T cell populations might be induced in response to different environmental, microbial and cytokine stimuli. Because of the dominant role of ILCs and γδ T cells in mucosal IL-22 production we used T-cell-reconstituted RAG2/IL-2RG mice to study the role of T-cell-produced IL-22 in mucosal inflammation. We found that IL-21 and AhR modulate the production of IL-22 by intestinal CD4+ T cells in vivo . In addition, it has been reported that the protective effects of some AhR dietary ligands in the DSS colitis model are T-cell-dependent, suggesting that IL-22 production by T cells plays a physiological role in the modulation of mucosal inflammation [54] . Additional support for this interpretation was recently provided by Basu et al . [29] , who described sequential waves of IL-22 production by ILCs and T cells responsible for host defence against Citrobacter rodentium infection. Indeed, it is possible that specialized ILCs with antigen-presenting cell activity participate in the induction and regulation of IL-22-producing mucosal T cells in vivo [55] . The study of the factors that control IL-22 production by different cell types is likely to identify appropriate targets for the therapeutic modulation of IL-22 production. A partial protection from DSS-induced colitis has been previously reported in complete, non-tissue-specific IL-21-deficient mice [56] . We believe that the differences in the role of IL-21 in DSS-induced colitis (protective in our work versus pathogenic in ref. 56 ) might reflect differential effects of IL-21 on ILCs and CD4+ T cells and the absence of ILCs in RAG2/IL2RG mice. Alternatively, these different outcomes might result from the use of IL-21-deficient mice in the work of Araki et al . [56] , instead of the IL-21R KO mice used in our studies. We found that AhR modulates IL-22 production by IL-22+ IL-17− T cells induced with IL-21, but AhR inhibition does not completely abrogate IL-22 production in vitro . Similar results have been recently reported for the role of AhR in the regulation of IL-22 production triggered in CD4+ T cells by IL-6 (ref. 28 ). Our data, however, suggest that AhR plays a more prominent role in the regulation of IL-22 production in vivo . A large proportion of intestinal IL-22+ T cells co-express IL-17, probably as a result of the local abundance of TGFβ1 which in combination with IL-6 and IL-21 favors the differentiation of Th17 cells that may control intestinal inflammation [8] , [57] . Indeed, our experiments using blocking antibodies indicate that TGFβ1 promotes AhR expression in IL-22-producing T cells. Th17 cells differentiated in the presence of TGFβ1 express higher amounts of AhR, and consequently AhR is a stronger regulator of IL-22 expression in Th17 cells than in IL-22+ IL-17− T cells [28] . Thus, the more prominent effects of AhR in the regulation of IL-22 in vivo might reflect the increased role of Th17 cells as a source of intestinal IL-22. It is also possible that local AhR ligands provided by the host, the diet or the commensal flora are more potent inducers of IL-22 expression in intestinal T cells. We and others have shown that AhR controls IL-22 and IL-10 production by Th17 (refs 20 , 22 , 23 ) and Tr1 (refs 35 , 43 , 58 ) cells. Considering the importance of IL-10 and IL-22 for the control of mucosal homeostasis and inflammation [2] , [3] , [59] , AhR seems to be closely linked to a transcriptional programme that limits immunopathology at environmental interfaces by the combined effects of IL-10 and IL-22. The regulation of AhR activity by endogenous, microbial, dietary and environmental ligands provides a molecular mechanism to adjust the mucosal production of IL-10 and IL-22. Moreover, it provides a potential target for therapeutic intervention. Mice Eight-week old C57BL/6 and double RAG2− IL-2RG-deficient female mice were purchased from the Jackson Laboratories. AhR-d-, IL21R- and ROR γ t-deficient mice were bred at Harvard Medical School, from breeders provided by the Jackson Laboratories. Mice were kept in a conventional, pathogen-free facility at the Harvard Institutes of Medicine. All mouse handling and in vivo experiments were carried out in accordance with guidelines prescribed by the Institutional Animal Care and Use Committee (IACUC) at Harvard Medical School. T-cell differentiation in vitro Naïve CD4+ T cells were stimulated with plate-bound antibodies against CD3 (145-2C11, 2 μg ml −1 ) and CD28 (PV-1, 2 μg ml −1 ), in the presence of IL-21 (30 ng ml −1 ) or IL-21 (30 ng ml −1 ) and IL-23 (30 ng ml −1 ) to generate Th22 cells; and IL-6 (30 ng ml −1 ), TGFβ1 (3 ng ml −1 ). Mouse IL-6, IL-21, IL-23 and TGFβ1 were purchased from R&D Systems. In some experiments we used TGFβ1-blocking antibodies at a final concentration of 10 μg ml −1 from R&D (Cat. no. AF-101-NA). FICZ was obtained from Enzo Life Sciences (PA, USA) and CH-223191 from EMD Chemicals (NJ, USA). We used an RPMI-based medium to minimize the activation of the cells by tryptophan-derived AhR ligands present in other tissue culture mediums [22] . RPMI was supplemented with 0.1 mM nonessential amino acids, 1 mM sodium pyruvate, L-glutamine (2 mM), penicillin (100 U ml −1 ), streptomycin (100 U ml −1 ), 10% heat-inactivated FBS (BioWhittaker, Inc.) and 2-mercaptoethanol. To evaluate the stability of IL-22-producing T cells induced with IL-21, in some experiments after an initial phase of activation in the presence of IL-21, T cells were re-stimulated with plate-bound antibodies to CD3 and CD28 for 48 h in the presence of medium, IL-21, TGFβ1 or TGFβ1and IL-6. Cytokine analysis Secreted cytokines were measured in supernatants of differentiated CD4+ T cells in vitro and in supernatants of colon samples ex vivo after 48 h by ELISA. For intracellular cytokine staining, cells were stimulated for 4 h at 37 °C in culture medium containing PMA (50 ng ml −1 ; Sigma, USA), ionomycin (1 μg ml −1 ; Sigma) and GolgiStop (1 μl ml −1 ; BD Biosciences, USA). After staining for the surface markers CD3 and CD4, cells were fixed and permeabilized using Cytofix/Cytoperm and Perm/Wash according to the manufacturer’s instruction (BD Biosciences, USA; eBioscience, USA). All antibodies were purchased from Biolegend and eBioscience. Data were acquired on a FACSCalibur (BD Biosciences) and analysed using the FlowJo software (Tree Star). qPCR RNA was extracted with RNAeasy columns (Qiagen, USA). cDNA was prepared using High Capacity cDNA Reverse Transcriptase kit following the manufacturer’s instructions (Applied Biosystems, USA) and used as template for real-time PCR. Probes were purchased from Applied Biosystems, and were used on the ViiA 7 Real-Time PCR System (Applied Biosystems). Expression was normalized to the expression of gapdh . The following probe mixtures were used: il1r (Mm01226962_m1), il6r (Mm00439653_m1), il21r (Mm00600319_m1), il23r (Mm00519942_m1), il10 (Mm0043614_m1), il17 (Mm00439619_m1), il21 (Mm00517640_m1), il22 (Mm00444241_m1), ahr (Mm01291777_m1), maf (Mm02581355_s1), rora (Mm01173766_m1), rorc (Mm00441144_g1), stat3 (Mm01219775_m1), foxp3 (Mm00475156_m1), socs3, mt1 (Mm00496660_g1), mt2 (Mm00809556_s1), gzma (Mm01304452_m1), gzmb (Mm00442834_m1), tbx21 (Mm00450960_m1) and gapdh (Mm99999915_g1). Gene expression analysis Transcriptome analysis was done using Affymetrix microarray MoGene_1_0_st on CD4+ T cells stimulated for 48 h in the presence of medium, IL-21 or IL-6 and TGFβ1. Microarray data were analysed using GeneSpring version12.5 software package (Agilent, Santa Clara, CA, USA). Samples were normalized using Quantile Normalization Algorithm. Fold change difference between IL-21-treated and untreated naïve CD4+ T cells was calculated to observe the differential expression profile of genes. Hierarchical clustering was performed on genes with fold change of ⩾ 1.5 using Euclidean distance metric to generate heat maps. We also performed principal component analysis to observe the separation between samples using GeneSpring version 7.3 software package (Agilent, Santa Clara, CA, USA). GEO: microarray data GSE55509. Western blot analysis Cells were lysed with RIPA buffer supplemented with protease inhibitor cocktail (Sigma, USA). Total T-cell lysates (20 μg) were resolved on 4–12% Bis-Tris Nupage gels (Invitrogen, USA) and transferred onto PVDF membranes (Millipore). The following primary antibodies were used: anti-AhR from Enzo Life Sciences (BML-SA210; 1/2,000 dilution); anti-RORγt from Abcam (Cat. no. 78007; 1/1,000 dilution) and anti-GAPDH from Cell Signalling Technology (Cat. no. 2111; 1/1,000 dilution). Western blot analysis was performed as described [60] and developed using SuperSignal West Femto Maximum Sensitivity Substrate, as instructed by the manufacturer (Pierce). Chromatin immunoprecipitation Cells were crosslinked with 1% paraformaldehyde and lysed with 0.35 ml of lysis buffer (1% SDS, 10 mM EDTA, 50 mM Tris–HCl, pH 8.1) containing 1 × protease inhibitor cocktail (Roche Molecular Biochemicals, USA). Chromatin was sheared by sonication and supernatants were collected after centrifugation and diluted in buffer (1% Triton X-100, 2 mM EDTA, 150 mM NaCl, 20 mM Tris–HCl, pH 8.1). Five micrograms of antibody were prebound for a minimum of 4 h to protein A and protein G Dynal magnetic beads (Invitrogen, USA) and washed three times with ice-cold PBS plus 5% BSA, and then added to the diluted chromatin and immunoprecipitated overnight. The magnetic bead–chromatin complexes were then washed three times in RIPA buffer (50 mM HEPES (pH 7.6), 1 mM EDTA, 0.7% Na deoxycholate, 1% NP-40, 0.5 M LiCl) followed by two times with TE buffer. Immunoprecipitated chromatin was then extracted with 1% SDS, 0.1 M NaHCO 3 and heated at 65 °C for at least 6 h to reverse the paraformaldehyde crosslinking. DNA fragments were purified with a QIAquick DNA purification Kit (Qiagen, USA) and analysed using SYBR green real-time PCR (Takara Bio Inc., USA). We used the following antibodies for ChIP: anti-pSTAT3 (Cat. no. 9132, Cell Signaling Technology, Inc., USA), anti-AhR (Cat. no. 9172, Cell Signaling Technology, Inc., USA), anti-cmaf (Cat. no. 9172, Cell Signaling Technology, Inc., USA), anti-Acetyl-H3 (Cat. no. 06-599, Millipore, MA, USA), Acetyl-H4 (Cat. no. 06-866, Millipore, MA, USA), anti-H3K4me3 (Cat. no. ab8580, Abcam, MA, USA), anti-H3K9me3 (Cat.no. ab8898, Abcam, MA, USA) and anti-H3K27me3 (Cat. no. 6002, Abcam, MA, USA). The primer pairs used in these experiments are listed in Supplementary Table 1 . Methyl-DNA immunoprecipitation The T cells were harvested after washing with PBS and genomic DNA was isolated using a DNeasy Blood and Tissue kit (Qiagen) and sheared by sonication to obtain DNA fragments of ~500 bp. Ten micrograms of sheared DNA were heated at 95 °C for 10 min and snap-chilled before mixing with 10 ul of freshly prepared protein A and protein G Dynal magnetic beads (Invitrogen) that were pre-incubated with 5 μg of either anti-5-methyl-cytidine antibody (Cat. no. ab10805) or mouse IgG control antibody (Cat. no. ab18413), both from Abcam, for a minimum of 4 h and washed three times with ice-cold PBS plus 5% BSA. The mixture was then incubated overnight in buffer (20 mM Tris–HCl (pH 8.1), 150 mM NaCl, 2 mM EDTA, 1% Triton X-100). The bead–DNA complexes were then washed three times in RIPA buffer (50 mM HEPES (pH 7.6), 1 mM EDTA, 0.7% Na deoxycholate, 1% NP-40, 0.5 M LiCl) followed by three times with TE buffer (10 mM Tris–HCl (pH 8.0), 1 mM EDTA). Immunoprecipitated DNA was then extracted by heating at 65 °C in 1% SDS, 0.1 M NaHCO 3 for at least 6 h. DNA fragments were purified with a QIAquick DNA purification Kit (Qiagen) and analysed using SYBR green real-time PCR. The primer pairs used in these experiments are listed in Supplementary Table 2 . Transfection and luciferase assays HEK293 cells were grown in DMEM supplemented with 10% fetal bovine serum, and transfected using the FuGENE HD (Roche, USA) transfection reagent according the manufacturer’s instructions. il22 promoter reporter construction was purchased from Dr Renauld (Ludwig Institute for Cancer Research and Experimental Medicine Unit, Universite Catholique de Louvain, Brussels, Belgium). Vectors coding for AhR and c-Maf were purchased from GeneCopoeia Inc (MD, USA), the vector coding for constitutively activated STAT3 was provided by Dr David Frank (Dana-Farber Cancer Institute, Boston, MA, USA). Firefly and renilla luciferase activity was analysed 48 h after transfection using a dual luciferase assay kit (Promega, USA). T-cell transfer and colitis induction Sorted splenic CD4+ T cells from C57BL/6, AhR-d and IL21R knock out mice were transferred i.p. (10 × 10 6 cells per mouse) into double RAG2− IL-2RG-deficient mice. One month after T-cell transfer, the recipient mice were checked for reconstitution of CD4+ T cells and colitis was induced with DSS. DSS (3%; MW: 36,000–50,000; MP Biomedicals, LLC) was dissolved in drinking water and administered for 7 days, and weight was monitored daily. Eight days after the initiation of the treatment with DSS the mice were killed, the colons were dissected and their length measured from the ileocecal junction to the anal verge. Histological evaluation of colitis Colonic tissue was removed and used for histologic evaluation by two independent investigators in a blinded fashion. The total histologic score represents the sum of non-ulcerative regions of epithelium and an infiltration score ranging from 0 to 6 as follows: epithelium: 0, normal morphology; 1, loss of goblet cells in small areas; 2, loss of goblet cells in large areas; infiltration: 0, no infiltration; 1, infiltration around crypt basis; 2, infiltration reaching the lamina muscularis mucosae; 3, extensive infiltration reaching the lamina muscularis mucosae and thickening of the mucosa with abundant oedema; 4, infiltration of the lamina submucosa. Ex viv o colon culture and ELISA Sections of 1 cm of the colon were excised, longitudinally halved and washed three times with sterile HBSS+HEPES medium (2% HEPES buffer, 1% penicillin–streptomycin and 0.05% gentamicin). The colon sections were placed into culture in complete Bruff’s media and cultured for 72 h at 37 °C with 5% CO 2 . The supernatants were harvested and the concentrations of IL-22 (Antigenix America), IL-6 and IL-23 (eBioscience) were determined by ELISA according to the manufacturer’s instructions. Statistical analysis Statistical analysis was performed using the Prism software (Graph Pad software, La Jolla, CA, USA). P <0.05 were considered statistically significant. How to cite this article: Yeste, A. et al . IL-21 induces IL-22 production in CD4+ T cells. Nat. Commun. 5:3753 doi: 10.1038/ncomms4753 (2014). Accession codes: Microarray data have been deposited in the GEO database under accession code GSE55509 .